The critical role of grain orientation and applied stress in nanoscale twinning Numerous recent studies have focused on the effects of grain size on deformation twinning in nanocrystalline fcc metals. However, grain size alone cannot explain many observed twinning characteristics. Here we show that the propensity for twinning is dependent on the applied stress, grain orientation and stacking fault energy. The lone factor for twinning dependent on grain size is the stress necessary to nucleate partial dislocations from a boundary. We use bulk processing of controlled nanostructures coupled with unique orientation mapping at the nanoscale to show the profound effect of crystal orientation on deformation twinning. Our theoretical model reveals an orientation-dependent critical threshold stress for twinning, which is presented in the form of a generalized twinnability map. Our findings provide a newfound orientation-based explanation for the grain size effect: as grain size decreases the applied stress needed for further deformation increases, thereby allowing more orientations to reach the threshold stress for twinning. Since the discovery that nanomaterials have a significantly higher propensity to twin than traditional metals [1] , [2] , [3] , [4] , [5] , [6] , several studies have been devoted to identifying the unconventional causes for twinning in these materials [7] , [8] , [9] , [10] , [11] . Many numerical and experimental works have shown that twinning occurs via different mechanisms in nanograined (NG) materials than in coarse-grained (CG) materials. In CG metals, twins nucleate by stress-driven defect reactions within the grain [12] , [13] , [14] , [15] . This nucleation mechanism permits several intersecting twins to form, potentially adversely affecting fracture behaviour [16] , [17] . Conversely, in NG metals, twins nucleate predominantly from reactions within grain boundaries [1] , [2] , [4] , [18] , [19] . With twins formed in this way, several desirable properties emerge, such as high strength, hardness, ductility and thermal stability, not seen in the CG counterparts [11] . With these exciting discoveries, fundamental studies have focused on identifying the effects of grain size on twinning in NG metals as grain size is decreased below 100 nm [9] , [11] , [20] . Generally, twins are not found in all grains even in NG materials comprised of homogeneous grain sizes [9] . Therefore, while having grain sizes of nanoscale dimensions may be important, it is not a sufficient condition for twinning, and it is clear that other key variables governing twinning need to be identified. In CG metals, the crystallographic orientation of the grain relative to the loading direction plays a major role in twinning [14] , [21] , [22] , [23] . This orientation effect is as strong as any grain size effect in CG metals. Two grains of the same size but different orientations have been observed to exhibit different twinnability [14] . With this in mind, the natural question to ask is, can the grain boundary-driven mechanism for twinning in nanomaterials invoke an orientation effect? Isolating grain-orientation effects in nanomaterials has been a much greater challenge than extracting grain size effects. With twins occurring heterogeneously and crystallographic orientations varying from grain to grain throughout the sample, data collected from a small number of grains are insufficient to prove orientation dependence. Extracting meaningful correlations between grain orientation and twinnability requires statistically significant sampling. Existing approaches cannot meet this requirement. Diffraction techniques (X-ray, neutrons) can detect global changes in orientation due to twinning, but cannot locally associate the twin with the grain orientation in which it was created. Traditional electron backscatter diffraction (EBSD) can make this correspondence but is limited to a practical spatial resolution of around 100 nm, which is not suitable for a NG study. Analyses using transmission electron microscopy can identify the parent grain orientation for a twin, but usually in a number of grains too small for sufficient statistics [9] , [24] . Even the recently developed technique of precession electron diffraction [25] , which can automatically map grain orientations at sufficient resolution, has not provided sufficient grain statistics for twinning correlations. Recently, we developed a novel, high spatial resolution EBSD technique through exploitation of a wedge-mounting scheme (WM-EBSD) that can resolve orientations in nanoscale-size grains and collect this data over hundreds of square microns of material [26] . WM-EBSD allows comparisons of twinning activity in grains of different orientations with these statistics inaccessible by other electron microscopy techniques. Advantageous for this study, rolling is a deformation mode in which a handful of crystal orientations are stable in many common fcc metals. These orientations have become a recognized standard and are designated as: brass (B), goss (G), copper (C), dillamore (D) and S [27] . Our neutron diffraction [28] and EBSD [28] measurements both confirm that these orientations develop in statistically significant amounts in the Cu layers made for this study before reaching the nanosize scales where twins begin to appear. We can now evaluate simultaneously the propensity to twin of many orientations of similar grain size and stress state. In this work we use WM-EBSD to examine orientation effects on deformation twinning in nanoscale Cu layers fabricated via severe plastic rolling deformation [28] . We discover that orientation has a profound effect on twinning at the nanoscale. We develop a theoretical model to explain the observed orientation effect, which is presented as a generalized twinnability map. Our analysis indicates that there is an orientation-dependent threshold stress above which a grain can twin. Measured twinning size dependence We apply WM-EBSD analysis to samples differing in average layer thickness, h , to examine the evolution of twinning with decreasing h . 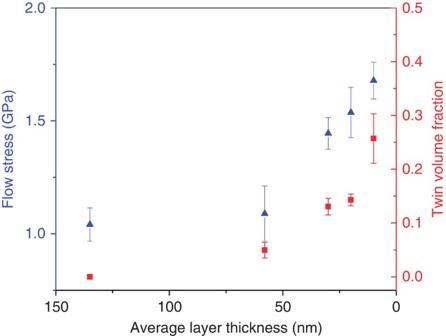Figure 1: Evolution of twin volume fraction and flow stress. Twin volume fraction (red squares) as a function of the average layer thickness. Flow stress values (blue triangles) are estimated from nanoindentation hardness values with error bars representing standard deviation. Flow stresses are included to illustrate how the material flow stress increases with decreasing average layer thickness. Figure 1 shows the evolution of twin fraction with average layer thickness. For average layer thicknesses below 500 nm, we have found that a single grain spans the layer thickness, and thus, layer thickness equals grain thickness [28] . We observe that twinning begins to appear at h =58 nm and continues to increase in volume fraction as h decreases to 30 nm and below. At 58 nm, grain dimensions in the transverse direction (TD) are generally greater than several hundred nanometres and rolling direction (RD) dimensions are greater than a micron, and it is estimated that the TD:ND (normal direction) grain aspect ratios are typically around 10:1 and the RD:ND aspect ratios are around 20:1 (ref. 28 ). Figure 1: Evolution of twin volume fraction and flow stress. Twin volume fraction (red squares) as a function of the average layer thickness. Flow stress values (blue triangles) are estimated from nanoindentation hardness values with error bars representing standard deviation. Flow stresses are included to illustrate how the material flow stress increases with decreasing average layer thickness. Full size image Measured twinning orientation dependence To examine the orientation dependence of twinning in these materials, we look at the statistical details of twinning for h =58 and 30 nm. The microstructural maps in Fig. 2 from the WM-EBSD technique provide a unique bird’s eye view of the nanostructure with the orientations simultaneously measured and designated by colour. The observed roughness is a visual effect from the wedge-mounting scheme that exaggerates asperities in the interface. In actuality, the interfaces are nearly planar and not as rough as they appear in Fig. 2 (ref. 26 ). The identification of twins and orientations is unaffected. 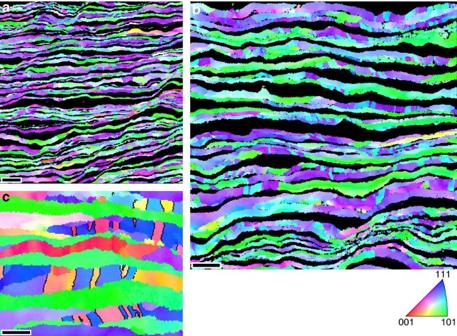Figure 2: Wedge section EBSD orientation maps. Composites (58 nm (a) and 30 nm (b)) showing Cu crystal directions parallel to the plate ND. (c) Detailed view of 30 nm composite showing Cu and Nb crystal directions parallel to the plate RD. Directions are indicated by the cubic standard triangle. The sectioning plane is at 10° to the ND and RD is horizontal. Scale bar, 2 μm (a), 1 μm (b) and 500 nm (c). Twinning statistics are generated from much larger EBSD scans than shown and are based on 6,815 Cu grains, 910 twinned grains and 2,022 twins for the 58-nm material and 1,711 Cu grains, 374 twinned grains and 1,476 twins for the 30-nm material. In both cases, the numbers of grains and twins analysed are unprecedented for nanomaterials. Figure 2: Wedge section EBSD orientation maps. Composites (58 nm ( a ) and 30 nm ( b )) showing Cu crystal directions parallel to the plate ND. ( c ) Detailed view of 30 nm composite showing Cu and Nb crystal directions parallel to the plate RD. Directions are indicated by the cubic standard triangle. The sectioning plane is at 10° to the ND and RD is horizontal. Scale bar, 2 μm ( a ), 1 μm ( b ) and 500 nm ( c ). Twinning statistics are generated from much larger EBSD scans than shown and are based on 6,815 Cu grains, 910 twinned grains and 2,022 twins for the 58-nm material and 1,711 Cu grains, 374 twinned grains and 1,476 twins for the 30-nm material. In both cases, the numbers of grains and twins analysed are unprecedented for nanomaterials. Full size image These images reveal that while most of the grains are the same size, some grains have twinned and others have not. The heterogeneity in twin formation is conventionally attributed to local stress fluctuations and the statistical nature of twinning [21] , [22] , [29] . Adopting a different viewpoint, we believe that the observed heterogeneity calls for statistically significant sampling to reveal meaningful microstructure/twin correlations. With several maps such as those in Fig. 2 totalling thousands of nanograins, orientation effects on twinning in the nanoscale regime are quantified for the first time. We use WM-EBSD to associate twins with the grain orientation in which they formed. 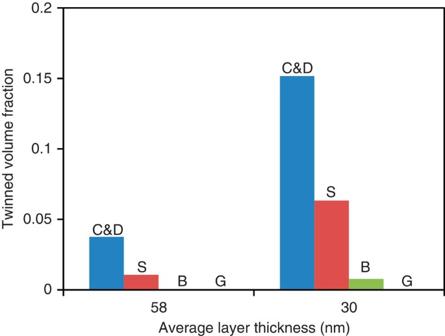Figure 3: Orientation dependence. Twinned volume fractions of several predominant Cu orientations. C, D, S, B and G refer to predominant orientations observed in the Cu in the present study. Figure 3 compares the twinned volume fractions for several Cu orientations obtained from thousands of Cu grains in the h =58 and 30 nm samples. The twinned volume fraction is the twinned area divided by the total grain area for each component. A 10° tolerance is used to define each orientation, and C&D orientations are grouped together because their orientations are separated by only 5°. The analysis reveals a definitive orientation dependence for twinning. Twinning is clearly most active in the C&D orientations and least active for B and G orientations. For S orientations, twinning activity increases considerably with decreasing average layer thickness. Figure 3: Orientation dependence. Twinned volume fractions of several predominant Cu orientations. C, D, S, B and G refer to predominant orientations observed in the Cu in the present study. Full size image Correlation of twinning with measured flow stress Figure 1 shows that the flow stress of our composite materials increases with decreasing layer thickness, where the flow stress is estimated as the nanohardness divided by 2.8 (ref. 30 ). This is consistent with the idea that the stress necessary to permanently deform a material increases with decreasing grain size [15] . Current twin nucleation models concede that high stresses promote twinning [31] . In this study, we also measure higher twin fractions for decreasing h ( Figs 1 and 3 ). However, by correlating twin fraction with orientation for h =58 and 30 nm, clear trends develop. First, the increase in twin fraction is because the same preferred orientations (C, D and S) form more twins ( Fig. 3 ). The non-preferred orientations, B and G, remain nearly free of twins. Thus, this analysis provides direct experimental evidence that the increase in twin volume fraction is not solely due to a grain size effect. Second, we see a considerable rise in the twin fraction within S orientations from 58 to 30 nm. This finding confirms that S is an orientation that promotes twinning, but that the stress required for twinning is larger than orientations C and D. Development of deformation twinning model To achieve a broad understanding beyond the orientations developed during rolling, we develop a theoretical model that predicts which nanosized grain orientations promote twinning under a given applied mechanical state. Our model has some similarities with other models used to explain size effects [20] and material property effects [32] in nanoscale metals. Primarily, these models are all based on the premise that the favourability of twinning is based on a competition between nucleation of a twinning partial and nucleation of a trailing slip partial dislocation [20] , [32] . In addition, our model considers some of the same forces acting on these dislocations [15] , [32] . Our analysis of this competition, our model geometry and our experimentally verified conclusions are unique. In fcc metals, such as Cu (and Ni, Al, Ag, Au), whether in a CG or NG form, a twin can form by the glide of lead partial dislocations with identical Burgers vectors on adjacent {111} planes [12] . Conversely, slip occurs in CG or NG materials when a lead partial dislocation is followed by a trailing partial dislocation on the same {111} plane [15] . A difference between CG metals and NG metals is that in NG metals the boundaries supply the partial dislocations needed for slip or twinning [1] , [2] , [4] , [18] , [19] . Molecular dynamics has shown that grain boundaries and even pristine phase boundaries can nucleate partial dislocations into Cu [33] , [34] . We propose that orientation affects the sequence of dislocation emissions from the boundary, and thus whether twinning or deformation slip predominates. Orientations in which the forces that drive twin nucleation are lower than those that drive slip dislocation nucleation favour twinning. 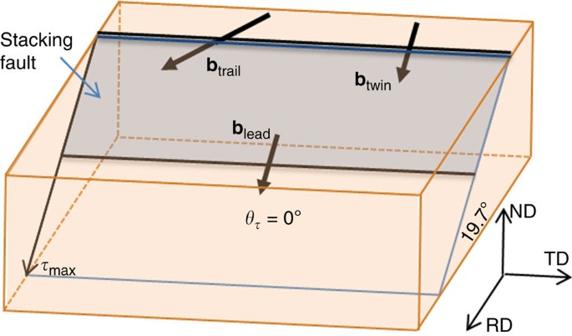Figure 4: Illustration of the slip/twin plane geometry relative to the specimen rolling geometry for C-oriented copper grains. A leading partial dislocation is emitted from a phase boundary (top surface) and trails a stacking fault along the slip/twin plane. Whether the driving force for twinning or slip is favoured depends on the magnitude ofτmaxand the angles between the direction ofτmaxand the potential twinning and trailing slip partial dislocation Burgers vectors. Specimen axes refer to the rolled plate ND, RD and TD. Figure 4 illustrates the influence of orientation on these critical forces. We assume that partial dislocations nucleate to supply work to the deforming crystal, and thus the partial that is first emitted, b lead , is the lead partial with the highest resolved shear stress. The grain orientation with respect to the stress state dictates the direction of τ max and θ τ , and the angle b lead makes with respect to τ max . Once b lead is selected, its equivalent b twin ( b twin has the same Burgers vector as b lead ) and the trailing b trail are known from crystallographic considerations. Although it is crystallographically possible for a twin to form through activation of other twinning partials at ±120° to the lead partial [24] , [35] , the large orientation dependence we observe and recent experiments revealing that zero-strain twinning is not dominant [35] are evidence that the twinning partials have the same Burgers vector as the lead, high Schmid factor partial dislocation. For a given orientation, the propensity to twin can be found by comparing the total force (per unit length) on b twin as it is emitted from the boundary, which is Figure 4: Illustration of the slip/twin plane geometry relative to the specimen rolling geometry for C-oriented copper grains. A leading partial dislocation is emitted from a phase boundary (top surface) and trails a stacking fault along the slip/twin plane. Whether the driving force for twinning or slip is favoured depends on the magnitude of τ max and the angles between the direction of τ max and the potential twinning and trailing slip partial dislocation Burgers vectors. Specimen axes refer to the rolled plate ND, RD and TD. Full size image with the force on b trail in the event it is emitted instead, which is where F int is the repulsive force exerted by b lead , (| b | τ max cos( θ τ )) and (| b | τ max cos( θ τ −60°)) are the force due to applied stress on the twinning dislocation and trailing dislocation, respectively, | b | is the magnitude of the partial dislocation Burgers vector, γ isf is the intrinsic stacking fault energy (SFE) (one layer) and γ esf is the two-layer SFE. Twinning becomes preferential when F twin > F trail or when where the inequality has been reorganized to emphasize the relationship of the parameters in Equation 3 with material properties, orientation and stress state. γ esf and | b | are material-dependent parameters. τ max contains an orientation dependency relating to how well the slip/twin plane is oriented relative to the bulk stress state, and θ τ contains an orientation dependency relating the Burgers vector directions to the direction of τ max . τ max is also dependent on the magnitude of the bulk applied stress. Here we use values calculated from ab initio density-functional theory (DFT) on Cu that give γ isf =36–41 mJ m −2 and γ esf =39–40 mJ m −2 (refs 36 , 37 ). A complete description of our model can be found in the Methods section. Development of twinnability map A significant implication emerging from this theoretical model is that orientations have a threshold stress above which they can twin. To better view this interdependence, in Fig. 5 we form a map of twinnability as a function of orientation and the macroscopic applied stress. The map shown in Fig. 5 is for γ esf =40 mJ m −2 and | b |=0.147 nm. The y axis, where τ max is normalized by σ Von Mises , represents how well the slip/twin plane is oriented relative to the bulk stress state. The x axis represents how well the lead/twinning Burgers vector is oriented relative to τ max . The contours represent the stress magnitude for which twinning becomes favourable for different combinations of slip/twin plane orientation and Burgers vector orientation. σ Von Mises was chosen as a scalar representation of a general stress state. 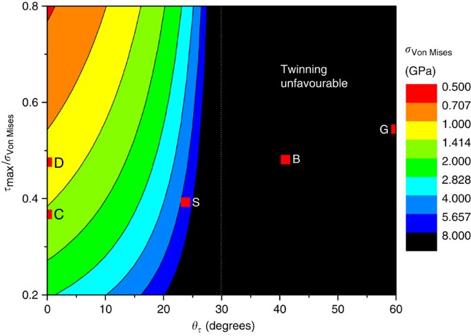Figure 5: Generalized twinnability map. Theyaxis, whereτmaxis normalized byσVon Mises, represents how well the slip/twin plane is oriented relative to the bulk stress state. Thexaxis,θτ, represents how well the lead/twinning Burgers vector is oriented relative toτmax. The contours represent the stress magnitude for which twinning becomes favourable for different combinations of slip/twin plane orientation and Burgers vector orientation.σVon Miseswas chosen as a scalar representation of a general stress state. The letters on the graph refer to the predominant orientations observed in this study.γesf=40 mJ m−2and |b|=0.147 nm. Figure 5: Generalized twinnability map. The y axis, where τ max is normalized by σ Von Mises , represents how well the slip/twin plane is oriented relative to the bulk stress state. The x axis, θ τ , represents how well the lead/twinning Burgers vector is oriented relative to τ max . The contours represent the stress magnitude for which twinning becomes favourable for different combinations of slip/twin plane orientation and Burgers vector orientation. σ Von Mises was chosen as a scalar representation of a general stress state. The letters on the graph refer to the predominant orientations observed in this study. γ esf =40 mJ m −2 and | b |=0.147 nm. Full size image In the upper left-hand corner of Fig. 5 , the slip/twin plane is well oriented resulting in a large value for τ max and the lead/twinning partial Burgers vector is at a small angle to τ max resulting in a lower threshold for twinning. The predicted contours suggest that orientations that lie progressively further away from this corner have increasingly higher threshold stresses and are thus more difficult to twin. On the right side of the map (black region), twinning is unlikely for any stress. To assess the validity of the map in Fig. 5 , we locate the five Cu orientations from this study on the map. The two orientations C and D in which twinning occurs at h =58 nm and below have the lowest threshold stresses. The S orientation has a higher threshold stress, which is consistent with the observation that twinning is less prevalent at 58 nm and then increases as the flow stress increases for h =30 nm. The B and G orientations, in which negligible amounts of twinning are observed, lie in the black regime of Fig. 5 where twinning is unfavourable. Our model also predicts that this threshold stress is directly proportional to SFE, an intrinsic material property on the general planar fault energy curve. Therefore, a material with higher SFEs requires more stress to twin than one with lower SFEs. A comparison of experimental observations of twinning with DFT-calculated SFEs agrees with this trend; Ag ( γ isf =16 mJ m −2 and γ esf =12 mJ m −2 (ref. 37 )) twins easier than Cu ( γ isf =36 mJ m −2 and γ esf =40 mJ m −2 (ref. 37 )), both of which twin more easily than Al ( γ isf =112 mJ m −2 and γ esf =112 mJ m −2 (ref. 37 )). This result is also consistent with most twinnability measures put forward to date [32] , [37] , [38] , [39] . Figure 5 represents the dependencies of twinning on orientation and stress for Cu, but can be adapted to other fcc metals by multiplying the twinning stress by the SFE ratio (fcc SFE/Cu SFE). However, the dependencies of twinning on orientation and stress are the novel aspects of the map, not the dependencies on SFEs. In summary, using a unique, high-resolution orientation mapping technique, we discover that orientation has a profound effect on twinning at the nanoscale. The conclusions from our analysis provide a simple explanation of these orientation effects that is consistent with experiment. The model and experiments show that orientations have a threshold stress above which they can twin. The model is applicable to twinning in other nanostructured fcc metals (nanowires, nanolayers, nanocrystalline metals) and for other stress conditions. Since such nanostructures can be manufactured with different crystal orientations, our findings reveal another method for controlling the interface-mediated mechanisms that determine nanomaterial behaviour. Experimental In the present study, we examine orientation effects in NG copper layers in nanostructured composites. To invoke deformation twinning within nanosized crystals, we fabricate composite layered nanostructured materials via the accumulative roll-bonding (ARB) severe plastic deformation process [28] . Briefly, the ARB process consists of a repetitive sequence of cutting, cleaning, stacking and roll bonding sheets of polycrystalline 99.99% pure Cu and 99.97% pure Nb metal. The ARB material analysed in the present study did not undergo any annealing steps. Using this process, we can create bulk sheets (greater than 3 mm total thickness) of metal ranging in layer thicknesses from around 1 mm (2 individual layers) down to below 15 nm (nearly 250,000 individual layers). With this approach, we control the average grain thickness throughout the sample by controlling the imposed amount of strain. We examine twinning phenomena in Cu layers, Cu being a prototypical material that has been the focus of many prior nanomaterial twinning studies [4] , [5] . Samples with layer thicknesses greater than or equal to 30 nm were cut from the materials and mounted using the wedge-mounting technique [26] . In this configuration, the metallographic sampling plane is at ~10° to the plate ND and 80° to the TD. Even with the benefits of WM-EBSD, it is not possible to sample the finest twins in our material because of our finite step sizes and the spatial resolution limits of EBSD, and it is estimated that the finest twins we are able to sample are around 10–20 nm thick. However, WM-EBSD does allow comparisons of twinning activity in grains of different orientations with these statistics inaccessible by other electron microscopy techniques. In addition, the finest twins contribute little to the measured volume fractions, and thus to the compared twinning activities. Samples with layer thicknesses <30 nm were mounted in plan view where the metallographic sampling plane is parallel to the ND. It is not possible to obtain grain thickness information from the plan-view specimens, but the continued texture evolution can be measured from which twin fraction estimates can be made. Metallographic samples were mechanically ground and polished finishing with vibratory polishing with 0.05 μm colloidal silica [28] . EBSD was performed on an FEI Inspect F using an accelerating voltage of 10 kV, a 50-μm aperture and a spot size of 4 with the scan of the 58-nm sample using a 50-nm step size and the 30-nm material using a 20-nm step size. EBSD data were collected using a TSL/EDAX system and initial data analysis was performed using TSL/EDAX OIM Analysis Software. Data post processing and twinning statistical analysis took advantage of a Los Alamos National Laboratory developed computer program [40] . Twinning model The propensity for twinning depends on the competition between available slip and twinning modes. FCC metals represent a special case where both slip and twinning take place on {111} planes and the twinning dislocations have the same Burgers vectors as the leading Shockley 1/6{112} partial dislocations [15] . For slip-dominated deformation, a leading Shockley 1/6<112> partial dislocation is nucleated from a boundary and is ultimately followed by a trailing partial dislocation on the same slip plane. The leading and trailing partial Burgers vectors sum to make a full ½<110> Burgers vector. For twinning, the same leading Shockley partial dislocation is ultimately followed by a twinning Shockley partial on an adjacent slip/twin plane. The competition between deformation twinning and dislocation slip in NC metals is, thus, the competition between the nucleation of a twinning partial and a trailing partial [20] , [32] . For both slip and twinning, the leading partial dislocation with the highest resolved shear stress nucleates from the boundary and trails a stacking fault (grey area in Fig. 4 ) in the slip plane as it glides into the grain. Grain aspect ratio measurements show that grains are significantly longer in the dislocation line direction compared with the ND grain dimension. Increases in line length due to dislocation deposition at the ends of the grains are, therefore, ignored. Once the leading partial has nucleated, whether slip or twinning occurs depends on whether the leading partial is followed by a trailing partial or twinning partial. The force per unit length acting to nucleate either a trailing partial or twinning partial is given by F rep is the elastic repulsion due to the leading partial dislocation and will be shown to be the same for either a trailing or twinning partial. F f is the force resulting from the change in fault energy due to the trailing or twinning dislocation. For a trailing partial, F f / L is positive and equal to the intrinsic SFE, γ isf . When a twinning dislocation nucleates on a plane adjacent to the leading dislocation, the twinning dislocation converts the single-layer, intrinsic stacking fault into a two-layer, extrinsic stacking fault with energy, γ esf , contributing to an additional force on the twinning dislocation equal to γ esf − γ isf . F τ is the force on the dislocation due to the applied stress and is equal to | b | τ max cos θ , where θ is the angle between the maximum shear stress and the Burgers vector. Therefore, In equations 5 and 6 we assume that the twinning dislocation has the same Burgers vector as the leading partial, and the trailing partial is the trailing partial with the highest resolved shear stress and is at 60° to the leading partial. Equation 6 for the force on the twinning dislocation also assumes that the height difference in the twinning dislocation plane and leading partial plane is negligible. These equations ignore dislocation character and other forces acting on the nucleating partial dislocations, such as elastic interactions with the neighbouring grains, which we assume are the same for both a trailing and twinning dislocation. F rep depends on the spacing of the lead partial relative to the trailing/twinning partial. The forces acting on the leading partial dislocation determine the spacing of the dislocation from the boundary and again include forces due to the applied stress, a restorative force due to the stacking fault, and elastic interactions with the emitting boundary and boundary on the opposite side of the grain. Assuming the elastic repulsion from the emitting boundary is the elastic interaction due to a twinning/trailing dislocation, and neglecting the elastic interaction with the opposite boundary results in an equilibrium spacing given by This gives a spacing of the lead dislocation at the moment when the twinning/trailing dislocation nucleates: For a twinning dislocation θ 2 = θ 1 and for a trailing dislocation θ 2 = θ 1 −60° The repulsive force on the twinning/trailing dislocation due to the lead dislocation is given by Substituting for r from above and taking θ 2 = θ 1 for a twinning dislocation and θ 2 = θ 1 −60° for a trailing dislocation: for both the cases of the twinning and trailing dislocation. Twinning becomes favourable when the driving force for nucleation of a twinning partial is greater than the driving force for nucleation of a trailing partial, or when Equation 6 is greater than Equation 5. Since F rep is the same for either a trailing or twinning dislocation, twinning becomes favourable when This can be rearranged to highlight orientation, stress and material property differences as How to cite this article: McCabe, R. J. et al . The critical role of grain orientation and applied stress in nanoscale twinning. Nat. Commun. 5:3806 doi: 10.1038/ncomms4806 (2014).